Primitive macrophages control HSPC mobilization and definitive haematopoiesis In vertebrates, haematopoietic stem/progenitor cells (HSPCs) first emerge in the aorta–gonad–mesonephros (AGM) before colonizing transitory and subsequently definitive haematopoietic organs allowing haematopoiesis throughout adult life. Here we identify an unexpected primitive macrophage population accumulated in the dorsal mesenteric mesoderm surrounding the dorsal aorta of the human embryo and study its function in the transparent zebrafish embryo. Our study reveals dynamic interactions occurring between the HSPCs and primitive macrophages in the AGM. Specific chemical and inducible genetic depletion of macrophages or inhibition of matrix metalloproteinases (Mmps) leads to an accumulation of HSPCs in the AGM and a decrease in the colonization of haematopoietic organs. Finally, in vivo zymography demonstrates the function of primitive macrophages in extracellular matrix degradation, which allows HSPC migration through the AGM stroma, their intravasation, leading to the colonization of haematopoietic organs and the establishment of definitive haematopoiesis. Blood cells are continuously produced from self-renewing progenitors with multi-lineage differentiation potential, called haematopoietic stem/progenitor cells (HSPCs). In vertebrates, haematopoiesis occurs as two waves. The ‘primitive’ wave produces only myelo-erythroid cells, whereas the ‘definitive’ wave gives rise to HSPCs [1] , [2] , [3] , [4] . In zebrafish, from 16 hours post fertilization (h.p.f. ), primitive haematopoietic cells produce macrophages and neutrophils that initiate innate immunity [5] , [6] , [7] . Zebrafish first HSPCs appear in the aorta–gonad–mesonephros (AGM), between the dorsal aorta (DA) and the posterior cardinal vein (PCV) by 30 h.p.f. (refs 3 , 8 ) where they start to express cd41 marker [9] . These HSPCs originate from aortic endothelial cells [10] , [11] through a process called endothelial haematopoietic transition or EHT [11] . Live imaging of mouse embryo sections [12] , cell sorting and differentiation experiments in human embryo have shown haemogenic endothelial cells to be at the immediate origin of haematopoietic cell clusters sprouting from the ventral side of the aorta [13] , which suggest that this process is conserved throughout evolution. We have previously documented that zebrafish HSPCs migrate from the AGM, enter the circulation and colonize the caudal haematopoietic tissue (CHT), analogous to the mammalian fetal liver. There they proliferate before colonizing the definitive haematopoietic organs, thymus and kidney [9] . HSPCs emerging between 30 and 55 h.p.f. give rise to all mature blood cell populations, including the second wave of macrophages. Macrophages from the first and second waves of haematopoiesis play important roles in development, tissue homeostasis [14] , innate and adaptive immunity and wound healing. In adults, they are also involved in the pathologies including chronic diseases [15] and cancer metastasis [16] , [17] . Macrophage-related processes are associated with their ability to migrate throughout the body and remodel surrounding stroma [18] by degrading the extracellular matrix (ECM) via the secretion of matrix metalloproteinases (MMPs for human and Mmps for zebrafish) and cathepsins [19] . MMPs have been shown to play important roles in tissue remodelling, or pathological processes [20] , especially MMP-2, 9 and 13. In zebrafish embryos, Mmp-9 and 13a are expressed by myeloid cells from 19 h.p.f. (refs 21 , 22 ). In this study, we imaged the accumulation of primitive macrophages in the AGM of both human and zebrafish embryos and analysed their interactions with emerging HSPCs. We demonstrated that primitive macrophages play a major role in the establishment of definitive haematopoiesis by permitting HSPC mobilization and colonization of haematopoietic organs via Mmps secretion and ECM remodelling. Macrophages accumulate in AGM during HSPC emergence Human HSPCs emerge between the 27th and the 40th day of development in the AGM as clusters of CD34+CD45+ cells adhering to the ventral wall of the DA [23] . Immunohistochemistry in human embryos at 34 days of development ( n =2) showed an intriguing accumulation of CD68+ macrophages in the mesenchyme beneath the ventral part of the CD34+ aortic endothelium ( Fig. 1a–a′′ ) and in the HSPC containing intra-aortic clusters ( Fig. 1b′ ). The number of macrophages in these locations, increased between 26 and 37 days of gestation, that is, in concomitance with the emergence of HSPCs ( Supplementary Fig. 1 ; n =3). 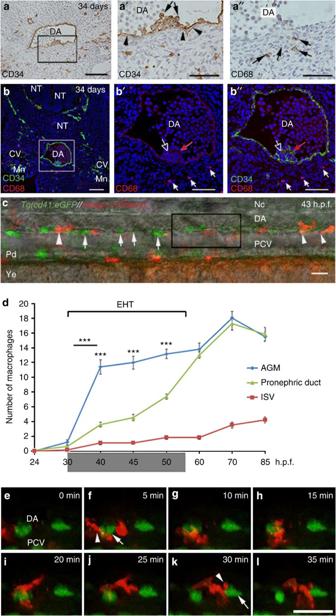Figure 1: Accumulation of macrophages in the AGM at the onset of definitive haematopoiesis. (a–b′′) Immunostained transverse sections of AGM region in 34-day human embryos (n=2). (a,a′,b,b′′) CD34 labels position of aortic endothelium (arrowhead) and HSPCs (a′, asterisks and arrows). (a′–a′) Higher magnification ofa, black box. CD68 stains macrophages (a′′,b′, arrow). (b′′) Higher magnification ofb, white box. Double CD34/CD68 immunofluorescence shows accumulation of macrophages (arrow and empty arrow), respectively, in the ventral wall of the DA and in HSPCs intra-aortic clusters (red arrow). (c) Maximum projection of confocalz-stack acquisitions in aTg(cd41:eGFP//mpeg1:mCherry)zebrafish embryo at 43 h.p.f. (10 μm depth); bright field is merged with green and red fluorescence. HSPCs/cd41:eGFP+ (arrow) and macrophages/mpeg1:mCherry (arrowhead) accumulate between the DA and the PCV. (d) Graph representing the specific accumulation of macrophages in the AGM during EHT compared with macrophages present in the intersomitic vessels and in pronephric ducts area. Data are shown as average ±s.e.m,n=20 (from two independent experiments).Pvalues are calculated for the difference between AGM and both intersomitic vessels and pronephric duct area at 40, 45 and 50 h.p.f. and for the difference of macrophage number in the AGM between 30 and 40 h.p.f. (underlined asterisks). ***P<0.001 (Kruskal–Wallis test for the whole evaluation and Student’st-test followed by Holm’s multiple comparison for individual stages). (e–l) Time-lapse confocal imaging ofTg(cd41:eGFP//mpeg1:mCherry)zebrafish embryo at 43 h.p.f. (higher magnification ofc, black box). (f–j) A macrophage (arrowhead) actively patrols in the AGM around a HSPC/cd41:eGFP+ (arrow) for 20 min, before heading toward another HSPC/cd41:eGFP+ (k,l). CV, cardinal vein; DA, dorsal aorta; ISV, intersomitic vessels; Mn, mesonephros; Nc, notochord; NT, neural tube; PCV, posterior cardinal vein; Pd, pronephric ducts; Ye, yolk extension. Scale bars, 50 μm (a,b′,b′′), 25 μm (a′,a′′,c,e–l), and 100 μm (b). See alsoSupplementary Fig. 1andSupplementary Movies 1 and 2. Figure 1: Accumulation of macrophages in the AGM at the onset of definitive haematopoiesis. ( a – b′′ ) Immunostained transverse sections of AGM region in 34-day human embryos ( n =2). ( a , a ′, b , b′′ ) CD34 labels position of aortic endothelium (arrowhead) and HSPCs ( a′ , asterisks and arrows). ( a ′– a′ ) Higher magnification of a , black box. CD68 stains macrophages ( a′′ , b′ , arrow). ( b′′ ) Higher magnification of b , white box. Double CD34/CD68 immunofluorescence shows accumulation of macrophages (arrow and empty arrow), respectively, in the ventral wall of the DA and in HSPCs intra-aortic clusters (red arrow). ( c ) Maximum projection of confocal z -stack acquisitions in a Tg(cd41:eGFP//mpeg1:mCherry) zebrafish embryo at 43 h.p.f. (10 μm depth); bright field is merged with green and red fluorescence. HSPCs/cd41:eGFP+ (arrow) and macrophages/mpeg1:mCherry (arrowhead) accumulate between the DA and the PCV. ( d ) Graph representing the specific accumulation of macrophages in the AGM during EHT compared with macrophages present in the intersomitic vessels and in pronephric ducts area. Data are shown as average ±s.e.m, n =20 (from two independent experiments). P values are calculated for the difference between AGM and both intersomitic vessels and pronephric duct area at 40, 45 and 50 h.p.f. and for the difference of macrophage number in the AGM between 30 and 40 h.p.f. (underlined asterisks). *** P <0.001 (Kruskal–Wallis test for the whole evaluation and Student’s t -test followed by Holm’s multiple comparison for individual stages). ( e – l ) Time-lapse confocal imaging of Tg(cd41:eGFP//mpeg1:mCherry) zebrafish embryo at 43 h.p.f. (higher magnification of c , black box). ( f – j ) A macrophage (arrowhead) actively patrols in the AGM around a HSPC/cd41:eGFP+ (arrow) for 20 min, before heading toward another HSPC/cd41:eGFP+ ( k , l ). CV, cardinal vein; DA, dorsal aorta; ISV, intersomitic vessels; Mn, mesonephros; Nc, notochord; NT, neural tube; PCV, posterior cardinal vein; Pd, pronephric ducts; Ye, yolk extension. Scale bars, 50 μm ( a , b ′, b′′ ), 25 μm ( a′ , a′′ , c , e – l ), and 100 μm ( b ). See also Supplementary Fig. 1 and Supplementary Movies 1 and 2 . Full size image We took advantage of zebrafish embryo remarkable optical properties to study the possible role of these macrophages during definitive haematopoiesis. In vivo imaging of Tg ( cd41:eGFP//mpeg1:mCherry) zebrafish embryos at 43 h.p.f. (green HSPCs and red macrophages) showed a similar accumulation of primitive macrophages along the entire length of the trunk in the direct vicinity of the ventral wall of the DA ( Fig. 1c ). Macrophage quantification confirmed their tissue-restricted accumulation in zebrafish AGM compared to surrounding tissues ( Fig. 1d , n =20). Interestingly, this accumulation was concomitant with HSPC/cd41:eGFP+ emergence in the AGM between 30 and 55 h.p.f. (ref. 11 ). Macrophages actively patrol in the AGM To assess if macrophages play a role in HSPC emergence, we imaged the behaviour of HSPCs and macrophages in Tg ( cd41:eGFP//mpeg1:mCherry) zebrafish embryos at 43 h.p.f. ( Fig. 1e–l ). As previously described, endothelial cells from the ventral wall of the aorta first bend then egress into the subaortic space to become free HSPCs [11] . At this stage, we observed that macrophages ( Fig. 1f ) continuously patrolled between the DA and the PCV, and intimately interacted with emerging HSPCs/cd41:eGFP+ ( Fig. 1e–l , Supplementary Movies 1 and 2 ). Live imaging of Tg(cd41:eGFP//mpeg1:mCherry) zebrafish embryo at 55 h.p.f. showed a macrophage/mpeg1:mCherry+ migrating in the AGM around an HSPC/cd41:eGFP+ during 32 min, before joining the PCV ( Supplementary Movie 2 , time code 00:56 to 1:00). This HSPC/cd41:eGFP+ would then join the PCV following the same route ( Supplementary Movie 2 ). A quantification of 112 HSPCs/cd41:eGFP+ (from 12 embryos) in the AGM revealed that 95.6% of them directly interacted with macrophages suggesting that macrophages could play an important role in emergence of HSPCs in the AGM. Macrophages are essential for definitive haematopoiesis To characterize their role in HSPC emergence, we chemically and genetically depleted primitive macrophages before or during definitive haematopoiesis at 25 and 45 h.p.f., respectively (before maturation of the second wave of macrophages). Liposome encapsulated clodronate ( L -clodronate) has been widely used to specifically induce the death of phagocytic macrophages in vitro and in vivo in mice and recently in zebrafish [24] , [25] . We first set about testing its efficiency, toxicity and specificity. Injection of 5 nl of L -clodronate stock suspension into the vein was sufficient for thorough macrophage depletion in embryos between 25 and 96 h.p.f. ( Supplementary Fig. 2b , n =200), compared with control embryos injected with PBS liposomes (L-PBS; Supplementary Fig. 2a , white arrows, n =25). The fate of macrophages in the AGM and in the CHT was examined during 18 h after L-clodronate injection. This revealed the steady decrease to complete disappearance of macrophages while passing through vacuolization and fragmentation ( Supplementary Fig. 2g ). No toxic effect was noticed on blood vessel organization ( Supplementary Fig. 2c,d , Tg(kdrl:caax:mCherry), n =15) nor on the evolution ( Supplementary Fig. 2h ), differentiation and function of primitive wave neutrophils [5] , the other myeloid cell population present in the embryo at this stage of development ( Supplementary Fig. 2e,f , arrow, Tg(mpx:eGFP), n =35). To evaluate the effect of macrophage depletion on HSPC emergence ( Fig. 2a–d ), we injected L-clodronate in Tg ( cd41:eGFP) embryos at 25 h.p.f. and observed that macrophage depletion did not prevent HSPCs/cd41:eGFP+ emergence in the AGM ( Fig. 2b versus a ), but led instead to their accumulation at 48 h.p.f. ( Fig. 2n , +60%, n =20). Whole-mount in situ hybridization (WISH) of c-myb confirmed the unaffected HSPC emergence in the AGM ( Fig. 2d versus c ). By contrast, macrophage depletion led to a very substantial decrease in the number of HSPCs/cd41:eGFP+ colonizing the CHT ( Fig. 2g,h versus e,f and n ; −89%, n =28) and the thymus at 72 h.p.f. ( Fig. 2l, versus k and n ; −91%, n =28), while injecting L-clodronate at 45 h.p.f. ( Fig. 2i ) caused less marked effects (−72% in CHT: Fig. 2j,n , n =28; and −50% in the thymus: Fig. 2m,n , n =22). The partial colonization observed after late L-clodronate injections was likely due to HSPCs that had already left the AGM before macrophage depletion. It further proved that L-clodronate was not toxic for HSPCs ( Fig. 2j ). 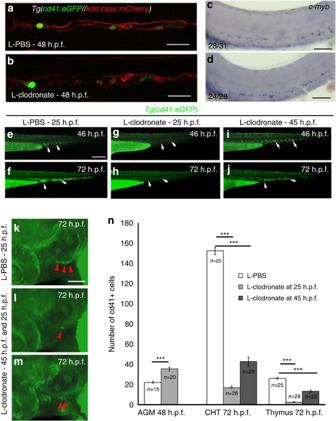Figure 2: Depletion of primitive macrophages reduces CHT and thymus colonization. (a,b) Macrophage depletion by L-clodronate injection at 25 h.p.f. does not affect HSPC/cd41:eGFP+ emergence in the AGM (48 h.p.f.). (c–d) WISH ofc-mybshows normal HSPC emergence in the AGM after macrophage depletion (N=21±0.72,n=15) compared with control embryos (N=14.9±0.51,n=15;P<0.001; Wilcoxon test).Nstands for the number ofc-mybcells per embryo,nfor the number of embryos. (e–m) Macrophage depletion by L-clodronate injection at 25 or 45 h.p.f. decreases HSPC/cd41:eGFP colonization at 46 and 72 h.p.f. of the CHT (g–j, white arrow) and thymus (l–m, red arrowhead) compared with control injected with L-PBS (e,f,k). (n) Macrophage depletion by L-clodronate injection at 25 h.p.f. causes HSPC/cd41:eGFP+ accumulation in the AGM at 48 h.p.f. (left column, +60%), while injection at 25 or 45 h.p.f. substantially reduces HSPC/cd41:eGFP+ colonization of the CHT at 72 h.p.f. (−89 and −72%, respectively) and thymus colonization at 72 h.p.f. (−91 and −50%, respectively) compared with the control injected with L-PBS. Data are shown as average ±s.e.m. ***P<0.001 (Wilcoxon test),n=number of embryos of minimal three independent experiments. Scale bars, 30 μm (a,b), 100 μm (c,d,k–m) and 250 μm (e–j). See alsoSupplementary Fig. 2. Figure 2: Depletion of primitive macrophages reduces CHT and thymus colonization. ( a , b ) Macrophage depletion by L-clodronate injection at 25 h.p.f. does not affect HSPC/cd41:eGFP+ emergence in the AGM (48 h.p.f.). ( c – d ) WISH of c-myb shows normal HSPC emergence in the AGM after macrophage depletion ( N =21±0.72, n =15) compared with control embryos ( N =14.9±0.51, n =15; P <0.001; Wilcoxon test). N stands for the number of c-myb cells per embryo, n for the number of embryos. ( e – m ) Macrophage depletion by L-clodronate injection at 25 or 45 h.p.f. decreases HSPC/cd41:eGFP colonization at 46 and 72 h.p.f. of the CHT ( g – j , white arrow) and thymus ( l – m , red arrowhead) compared with control injected with L-PBS ( e , f , k ). ( n ) Macrophage depletion by L-clodronate injection at 25 h.p.f. causes HSPC/cd41:eGFP+ accumulation in the AGM at 48 h.p.f. (left column, +60%), while injection at 25 or 45 h.p.f. substantially reduces HSPC/cd41:eGFP+ colonization of the CHT at 72 h.p.f. (−89 and −72%, respectively) and thymus colonization at 72 h.p.f. (−91 and −50%, respectively) compared with the control injected with L-PBS. Data are shown as average ±s.e.m. *** P <0.001 (Wilcoxon test), n =number of embryos of minimal three independent experiments. Scale bars, 30 μm ( a , b ), 100 μm ( c , d , k – m ) and 250 μm ( e – j ). See also Supplementary Fig. 2 . Full size image To fully validate the effect of macrophage depletion on haematopoietic organ colonization, we set inducible nitroreductase genetic depletion of macrophages [26] as an alternate experimental approach. Expression of E.coli nitroreductase under the control of mpeg1 promoter allows the inducible tissue specific and reversible depletion of macrophages by soaking embryos in the prodrug metronidazole. Similar to L-clodronate, metronidazole macrophage depleted embryos ( Fig. 3b versus a ) exhibited an impaired CHT colonization by HSPCs/cd41:eGFP+ ( Fig. 3b′ versus a′ , −68% at 60 h.p.f., Fig. 3c , n =24) as well as an accumulation of HSPCs/cd41:eGFP in the AGM ( Supplementary Fig. 3a , +71% at 60 h.p.f., n =11). Macrophages still present after 42 h of metronidazole treatment ( Fig. 3b ) result either from partial depletion or delayed depletion or both and most likely explain the partial CHT colonization by HSPC compared with embryos injected with L-clodronate ( Fig. 3b′ and Fig. 2g,h ). 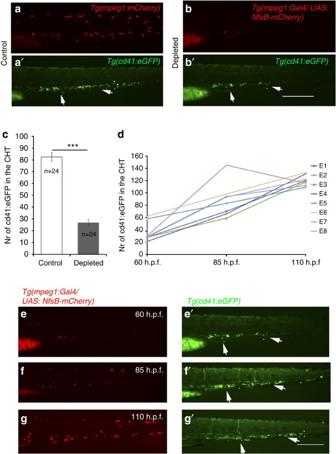Figure 3: Rescue of CHT colonization after macrophage reappearance. (a,b′) Metronidazole induced depletion of macrophages (a,b) results in the decrease of CHT colonization (a′,b′). (c) Metronidazole induced macrophage depletion substantially reduces HSPC/cd41:eGFP+ colonization of the CHT (−68%) at 60 h.p.f. compared with the controlTg(cd41:eGFP//mpeg1:mCherry)embryos treated with metronidazole. Data are shown as average ±s.e.m. ***P<0.001 (Wilcoxon test),n=number of embryos of minimal three independent experiments. (d) Rescue of CHT colonization is held due to metronidazole withdrawal at 60 h.p.f. Graph represents number of HSPCs/cd41:eGFP+ accumulated in the CHT at 60, 85 and 110 h.p.f. Data are shown as longitudinal study of single embryo,n=8. (e–g) Reappearance of macrophages is detected after the metronidazole wash-out during the following 2 days (25 (f) and 50 h post withdrawal (g)). The increasing number of HSPCs/cd41:eGFP+ accumulated in CHT (e′–g′) is directly connected to reappearance of macrophages in the embryo (e–g). Scale bar, 250 μm. See alsoSupplementary Fig. 3. Figure 3: Rescue of CHT colonization after macrophage reappearance. ( a , b′ ) Metronidazole induced depletion of macrophages ( a , b ) results in the decrease of CHT colonization ( a′ , b′ ). ( c ) Metronidazole induced macrophage depletion substantially reduces HSPC/cd41:eGFP+ colonization of the CHT (−68%) at 60 h.p.f. compared with the control Tg(cd41:eGFP//mpeg1:mCherry) embryos treated with metronidazole. Data are shown as average ±s.e.m. *** P <0.001 (Wilcoxon test), n =number of embryos of minimal three independent experiments. ( d ) Rescue of CHT colonization is held due to metronidazole withdrawal at 60 h.p.f. Graph represents number of HSPCs/cd41:eGFP+ accumulated in the CHT at 60, 85 and 110 h.p.f. Data are shown as longitudinal study of single embryo, n =8. ( e – g ) Reappearance of macrophages is detected after the metronidazole wash-out during the following 2 days (25 ( f ) and 50 h post withdrawal ( g )). The increasing number of HSPCs/cd41:eGFP+ accumulated in CHT ( e′ – g′ ) is directly connected to reappearance of macrophages in the embryo ( e – g ). Scale bar, 250 μm. See also Supplementary Fig. 3 . Full size image As the genetic depletion is reversible by removing metronidazole from the medium, we measured macrophage reappearance during the 2 days following prodrug withdrawal ( Fig. 3d–g ) and its effect on haematopoiesis in the CHT ( Fig. 3d,e′ ). Indeed the number of HSPCs/cd41:eGFP+ accumulated in the CHT was directly correlated with both the reappearance of macrophages in embryos ( Fig. 3d and Supplementary Fig. 3b ) and the decrease of the HSPCs/cd41:eGFP accumulation in the AGM ( Supplementary Fig. 3a ). Altogether these results demonstrated the crucial role of macrophages in haematopoietic organ colonization. Mmps allow HSPC intravasation then organ colonization Various proteases, especially MMP-2 and -9 that share high similarity in protein sequence with their zebrafish orthologs (90 and 73%, respectively) [21] , [27] have been shown to be associated with ECM degradation and cell intravasation mediated by macrophages. To study the role of MMPs, Tg(cd41:eGFP) embryos were soaked from 38 h.p.f. in two different MMP inhibitors; GM6001, a general MMP inhibitor [28] or SB-3CT, a specific inhibitor of MMP-2 and 9 (Gelatinases A and B) [29] . This inhibition resulted in HSPCs/cd41:eGFP+ accumulation in the AGM at 60 h.p.f. ( Fig. 4e,f and Supplementary Fig. 4d , +26% and +51% for GM6001 and SB-3CT respectively) compared with control embryos ( Fig. 4d ), while it led to a consequent decrease in HSPCs/cd41:eGFP colonization of the CHT at 60 h.p.f. ( Fig. 4a–c ; −43 and −66% respectively, Supplementary Fig. 4d , n =42 and n =44) and the thymus at 72 h.p.f. ( Supplementary Fig. 4a–d , −44 and −75%; respectively, n =30 and 29). 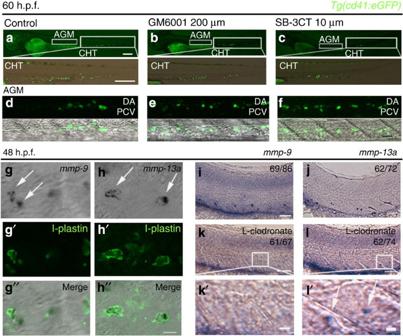Figure 4: Role of MMPs in HSPC mobilization and colonization of the CHT. (a–f) Inhibition of MMPs impairs HSPC mobilization and the colonization of CHT. (a) HSPCs are present inTg(cd41:eGFP)embryo at 60 h.p.f. (bottom, enlarged CHT). Small box shows the AGM imaged by confocal microscopy ind. (d) Green fluorescence shows the presence of cd41:eGFP cells in the AGM at 60 h.p.f. (bottom, merged with transmission channel). (b,c) Treatment with GM6001 (b,n=42) or SB-3CT (c,n=44) reduces CHT colonization by HSPCs/cd41:eGFP+ cells compared with control (a,n=45). (e,f) Confocal imaging of the AGM reveals accumulation of HSPCs/cd41:eGFP+ cells in AGM compared with the control (d) (d–f,n=23; three frames combined). Confocal imaging of WISH (g,h, arrows) combined with L-plastin immunofluorescence (green) (g′,h′) are merged ing′′andh′′. (i–l) WISH ofmmp-9(i) andmmp-13a(j) in the AGM in control embryos and after macrophage depletion by L-clodronate (k,l). Close-ups of macrophage depleted embryos ink′,l′(arrow). Scale bar, 250 μm (a–c), 30 μm (d–f), 50 μm (i–l), 10 μm (g,h′′,k′,l′). See alsoSupplementary Fig. 4. Figure 4: Role of MMPs in HSPC mobilization and colonization of the CHT. ( a – f ) Inhibition of MMPs impairs HSPC mobilization and the colonization of CHT. ( a ) HSPCs are present in Tg(cd41:eGFP) embryo at 60 h.p.f. (bottom, enlarged CHT). Small box shows the AGM imaged by confocal microscopy in d . ( d ) Green fluorescence shows the presence of cd41:eGFP cells in the AGM at 60 h.p.f. (bottom, merged with transmission channel). ( b , c ) Treatment with GM6001 ( b , n =42) or SB-3CT ( c , n =44) reduces CHT colonization by HSPCs/cd41:eGFP+ cells compared with control ( a , n =45). ( e , f ) Confocal imaging of the AGM reveals accumulation of HSPCs/cd41:eGFP+ cells in AGM compared with the control ( d ) ( d – f , n =23; three frames combined). Confocal imaging of WISH ( g , h , arrows) combined with L-plastin immunofluorescence (green) ( g′ , h′ ) are merged in g′′ and h′′ . ( i – l ) WISH of mmp - 9 ( i ) and mmp - 13a ( j ) in the AGM in control embryos and after macrophage depletion by L-clodronate ( k , l ). Close-ups of macrophage depleted embryos in k ′, l ′ (arrow). Scale bar, 250 μm ( a – c ), 30 μm ( d – f ), 50 μm ( i – l ), 10 μm ( g , h′′ , k′ , l′ ). See also Supplementary Fig. 4 . Full size image We thus concluded that both primitive macrophages and Mmps secretion are essential for HSPC mobilization and consequently haematopoietic organ colonization. Mmp-9 and mmp-13a are expressed by macrophages To establish a direct connection between macrophages and mmps expression in the AGM, we combined L-plastin immunostaining (a leukocyte marker) with WISH of 48 h.p.f. embryos using mmp-2 , mmp-9 and mmp-13a probes. Mmp-9 and -13a expression patterns ( Fig. 4g–j ) matched to myeloid cells ( Fig. 4g′–h′′ , n =10) but not mmp-2 expression ( Supplementary Fig. 4e,f , n =10), which gave a broader pattern in the trunk region ( Supplementary Fig. 4e–e′′ ). As L-plastin is expressed by different myeloid populations, we analysed mmps expression in embryos injected with L-clodronate. We observed in the AGM that mmp-2 expression profile ( Supplementary Fig. 4g,g′ ) was unchanged after macrophage depletion while mmp-13a ( Figs 4l,l′ ) was significantly reduced and mmp-9 completely disappeared ( Fig. 4k,k′ ). We concluded that macrophages expressing mmp-9 are unambiguously associated with HSPC mobilization and intravasation. Macrophage-mediated ECM degradation WISH showed that mmp-9 is expressed by primitive macrophages, but no direct demonstration was made of macrophage-mediated matrix degradation. We therefore decided to visualize matrix degradation by in vivo zymography [30] using gelatin as an intermediate product of collagen degradation. We injected highly quenched fluorescein-labelled gelatin (Gelatin-FITC) into the muscles of Tg(mpeg1:mCherry) embryos ( Fig. 5a , n =10). Degradation of this substrate releases FITC from its quencher resulting in green fluorescence. Specific punctiform green fluorescence was observed around spherical cells that appeared as unlabelled ghosts ( Fig. 5b,c , blue dots and arrow), while embryos soaked in MMP inhibitors did not show any FITC signal fluorescence ( Supplementary Fig. 5a–c , middle and right, Supplementary Movie 5 ) nor did L-clodronate injected embryos ( Supplementary Fig. 5d,e ). Time-lapse imaging showed co-localization of macrophage trails and emitted FITC fluorescence ( Fig. 5c′–f, j–m , Supplementary Movies 3–4 and Supplementary Fig. 5f , n =3, 79% of liberated FITC was correlated to macrophages). 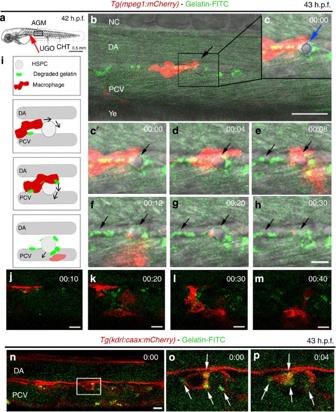Figure 5:In vivozymography shows macrophage-induced proteolysis of the ECM. (a) Drawing indicates the site of intramuscular injection of Gelatin-FITC (red arrow) and the area imaged inb(black box). (b–h)In vivoimaging of the AGM at 43 h.p.f. was carried out just after gelatin-FITC injection inTg(mpeg1:mCherry). Green staining indicates gelatin degradation after macrophage migration (red) inc–h(n=10). (c–h) Close-ups (b, black box) show a patrolling macrophage (red) that degrades gelatin (green dots), induces HSPC migration through the ECM (arrow), followed by intravasation (Supplementary movie 3). (c) Arrow shows unlabelled round cells corresponding to HSPCs (blue dots). (i) Schematic view of gelatin degradation by a red macrophage around a light gray HSPC in the AGM. First diagram shows macrophage migration around an HSPC. Macrophage migration results in green spots corresponding to gelatin degradation, followed by HSPC intravasation (f–h,Supplementary Movie 3). (j–m) Zoomed imaging shows two macrophages in the AGM-degrading Gelatin-FITC during their passage (Supplementary Movie 4). (n) Gelatin degradation is localized around an emerging HSPC/mCherry+ cell after injection of gelatin-FITC in aTg(kdrl:caax:mCherry)embryo. (o,p) Close-ups of emerging HSPC/mCherry+ intravasation in the vein (inset,n) after ECM degradation in 4 min. Time code in hours and minutes, upper right corner. White arrows point the FITC liberation next to the intravasating HSPC/mCherry+ cells. UGO, urogenital opening. Scale bars, 0.5 mm (a), 30 μm (b) and 10 μm (c′-n). See alsoSupplementary Fig. 5andSupplementary Movies 3–5. Figure 5i provides a schematic diagram of a macrophage migrating around the HSPC and leaving a trail of degraded gelatin ( Fig. 5c′–h , Supplementary Movie 3 ), followed by the migration and intravasation of a round cell between two spots of degraded gelatin ( Fig. 5f–h , arrow; Supplementary Movie 3 ). To confirm that these migrating round cells are HSPCs, we injected Gelatin-FITC into Tg(kdrl:caax:mCherry) embryos in which vascular endothelium and HSPCs express the mCherry protein [10] . We observed the same specific punctiform fluorescence around HSPCs/mCherry+ cells emerging from the wall of the aorta ( Fig. 5n–p , n =4). Figure 5: In vivo zymography shows macrophage-induced proteolysis of the ECM. ( a ) Drawing indicates the site of intramuscular injection of Gelatin-FITC (red arrow) and the area imaged in b (black box). ( b – h ) In vivo imaging of the AGM at 43 h.p.f. was carried out just after gelatin-FITC injection in Tg(mpeg1:mCherry) . Green staining indicates gelatin degradation after macrophage migration (red) in c – h ( n =10). ( c – h ) Close-ups ( b , black box) show a patrolling macrophage (red) that degrades gelatin (green dots), induces HSPC migration through the ECM (arrow), followed by intravasation ( Supplementary movie 3 ). ( c ) Arrow shows unlabelled round cells corresponding to HSPCs (blue dots). ( i ) Schematic view of gelatin degradation by a red macrophage around a light gray HSPC in the AGM. First diagram shows macrophage migration around an HSPC. Macrophage migration results in green spots corresponding to gelatin degradation, followed by HSPC intravasation ( f – h , Supplementary Movie 3 ). ( j – m ) Zoomed imaging shows two macrophages in the AGM-degrading Gelatin-FITC during their passage ( Supplementary Movie 4 ). ( n ) Gelatin degradation is localized around an emerging HSPC/mCherry+ cell after injection of gelatin-FITC in a Tg(kdrl:caax:mCherry) embryo. ( o , p ) Close-ups of emerging HSPC/mCherry+ intravasation in the vein (inset, n ) after ECM degradation in 4 min. Time code in hours and minutes, upper right corner. White arrows point the FITC liberation next to the intravasating HSPC/mCherry+ cells. UGO, urogenital opening. Scale bars, 0.5 mm ( a ), 30 μm ( b ) and 10 μm ( c′ - n ). See also Supplementary Fig. 5 and Supplementary Movies 3–5 . Full size image In vivo zymography therefore provided a final demonstration of matrix degradation in the AGM by macrophage secreted proteases followed by HSPC mobilization and vein intravasation. The studies described herein show an unexpected accumulation of primitive macrophages in the AGM region (ventrally to the DA) of human and zebrafish embryo. We previously reported that zebrafish HSPCs emerge in the subaortic mesenchyme then enter the PCV circulation through peculiar structures, which facilitate HSPC intravasation [9] . Live imaging in HSPC- cd41:eGFP+/ macrophage -mpeg1:mCherry+ zebrafish embryo shows these tiny entry points are created by macrophages during their migration through the stroma, which will allow HSPCs to join the PCV. Macrophage depletion at early stages of development (25 h.p.f.) prevents the colonization of haematopoietic organs without affecting EHT in the AGM, while late depletion (45 h.p.f.) leads to less pronounced effects. Because zebrafish definitive haematopoiesis occurs between 30 and 55 h.p.f. (ref. 3 ), the partial colonization observed after late depletion is likely due to HSPCs which had already left the AGM before macrophage depletion. We show here that these entry points are formed by Mmps-secreting macrophages. Specific chemical Mmps inhibition together with combined WISH and immunofluorescence staining established that macrophages are involved in HSPC mobilization via Mmp-9 secretion. Therefore, our data suggest that primitive macrophages play an essential role in definitive haematopoiesis by inducing Mmps-mediated degradation of the ECM around HSPC in the AGM region. Matrix degradation allows mobilization and migration of HSPC into the stroma, driving their intravasation into the vein, leading ultimately to the colonization of haematopoietic organs and the establishment of definitive haematopoiesis (as summarized in Fig. 6 ). 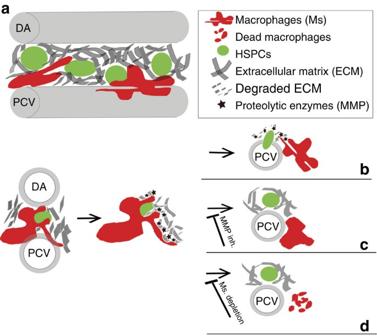Figure 6: Primitive macrophages in HSPC mobilization and definitive haematopoiesis. (a) Macrophages (red) interact with HSPCs (green) in the AGM during haematopoiesis. (b) ECM degradation by macrophages enables HSPC mobilization, intravasation and haematopoietic organ colonization. Mmps inhibition (c) or macrophage depletion (d) result in HSPC accumulation in the AGM. inh., inhibition. Figure 6: Primitive macrophages in HSPC mobilization and definitive haematopoiesis. ( a ) Macrophages (red) interact with HSPCs (green) in the AGM during haematopoiesis. ( b ) ECM degradation by macrophages enables HSPC mobilization, intravasation and haematopoietic organ colonization. Mmps inhibition ( c ) or macrophage depletion ( d ) result in HSPC accumulation in the AGM. inh., inhibition. Full size image Another intriguing observation of this report is that a specific accumulation of primitive macrophages is also detected in the human embryo. CD68+ macrophages are indeed concentrated in the mesenchyme beneath the ventral wall of the human embryonic aorta but also associated with the intra-aortic HSPC clusters. Even if, in the human, like any mammalian embryo the mobilization of HSPCs occurs within the DA circulation [1] , this accumulation of macrophages observed in the AGM, suggests that they could play a role in the establishment of definitive haematopoiesis also in these species. Therefore, we speculate that in human embryo, macrophages can facilitate the release of HSPCs from intra-aortic clusters, through a process evolutionary conserved. Recent findings have demonstrated that macrophages maintain HSCs in adult bone marrow niches and their depletion mobilizes HSPCs in the bloodstream [31] , [32] . Our data show that during development, macrophages may have the opposite function by mobilizing HSPCs from the AGM followed by their intravasation and colonization of haematopoietic organs. This mobilization involves ECM degradation by the local secretion of Mmps. Recent studies have shown that tumour-associated macrophages play a role in ECM remodelling in tumour stroma through the release of proteases from invadopodia, (mainly MMP-2 and 9) (ref. 18 , 19 ). These enzymes degrade the rigid stroma of tumours and enable CICs (cancer-initiating cells) to intravasate and seed secondary sites, that is, metastasis [33] . Our observations show marked similarities with this process, suggesting that HSPC and CIC migration might be comparable. It will thus be interesting to explore whether HSPCs also release factors that attract macrophages and what are their nature. Human tissues and immunostaining Human embryos were obtained from voluntary abortions performed according to guidelines and with the approval of the French National Ethics Committee. Patients gave their written consent for the embryos to be used for research purposes. Embryo sections (5 μm) were incubated with anti-CD34 (3.2 μg ml −1 , Miltenyi) or anti-CD68 (10 μg ml −1 , eBioscience) antibodies, then with biotinylated secondary antibodies (10 μg ml −1 , Immunotech) and with peroxidase-labelled streptavidin (0.6 μg ml −1 , Immunotech). Fluorescence-conjugated secondary antibodies (0.5 μg ml −1 , Biolegend) were used for double staining. Zebrafish transgenic lines and live imaging Wild-type AB, Tg(kdrl:Has.HRAS-mCherry) (here cited as kdrl:caax:mCherry ) [34] , Tg(cd41:eGFP) [35] , Tg(mpx:eGFP) [36] , Tg(mpeg1:mCherry-f) (here cited as mpeg1:mCherry ; see below) and Tg(mpeg1:Gal4FF//UAS-E1b:Eco.NfsB-mCherry) (here cited as mpeg1:GAL4//UAS:NfsB-mCherry ) [26] transgenic embryos were staged as described by Kimmel et al . [37] All experiments were carried out following the protocol CEEA-LR-13007 approved by the Animal Care and Use Committee Languedoc-Roussillon. Human and zebrafish embryos (lateral views, rostral to the left) were imaged on Leica SP5 confocal ( Fig. 1a–b′′ , Fig. 5 , Supplementary Fig. 1 and Supplementary Movies 3 and 4 ), Leica SPE confocal ( Fig. 1c ; Fig. 4d,g–h′′ and Supplementary Fig. 4a–c, e–e′′ , Supplementary Fig. 5d,e ), DeltaVision OMX (Applied Precision; Figs 1e–l and Supplementary Movie 1 ), Zeiss LSM510 confocal ( Fig. 2a,b , Supplementary Fig. 5a–c , Supplementary Movies 2 and 5 ), Zeiss V12 ( Fig. 2c,d , Fig. 3a–b′ and e–g′ ), Trophos Plate Runner ( Figs 2e–m ), Olympus MVX10 ( Fig. 4a–c and Supplementary Fig. 2a–f ) and Zeiss AxioImager Z.1 ( Fig. 4i–l ′ and Supplementary Fig. 4f–g′ ). Generation of mpeg1:mCherry-f transgenic Zebrafish line A 1.9-kb mpeg1 promoter fragment encompassing the mpeg sequences driving promoter activity specifically in macrophages [38] was amplified by PCR using following forward 5′- TTGGAGCACATCTGAC -3′ and NotI-introducing reverse 5′- TTATAGCGGCCGCGAAATGCTCTTGACTTCATGA -3′ primers. Resulting product was digested by NotI and ligated to farnesylated mCherry protein coding sequence so that Mpeg1 ATG initiation codon would be in frame with downstream mCherry-F cds in a Tol2 derived vector. The resulting plasmid was injected along with transposase mRNA in one cell stage zebrafish embryos to achieve germline integration. Macrophage chemical and inducible genetic depletion Macrophages were depleted by injecting 5 nl of L-clodronate into the caudal vein (gift from M. Daeron Laboratory). L-PBS was injected as a control. Embryos with L-clodronate aggregates causing vessel occlusions and shunts were discarded. Metronidazole-mediated depletion was performed by using double transgenic fish Tg(mpeg1:GAL4//UAS:NfsB-mCherry) [26] crossed with Tg(cd41:eGFP) to evaluate the effect of macrophage depletion on cd41+ cells. Embryos at 18 h.p.f. were treated with freshly prepared 10 mM metronidazole (Sigma) in 0.1% DMSO (dimethylsulphoxide) solution protected from light until the evaluation (60 h.p.f. ), then rinsed with embryo water. Tg(cd41:eGFP//mpeg1:mCherry ) embryos treated with 10 mM metronidazole were used as control. MMP inhibition assay Embryos were soaked in GM6001 (200 μM, Merck Millipore), SB-3CT (10 μM, Enzo Life Sciences) or DMSO (0.2%) as a control from 38 h.p.f. until observation. WISH and immunofluorescence staining WISH was performed according to Thisse ( http://zfin.org/zf_info/zfbook/chapt9/9.82.html ). Embryos at 48 h.p.f. were fixed, dehydrated with methanol, digested with proteinase K (New England Biolabs) and fixed again. Prehybridization was performed at 68 °C in HM+ buffer (50% formamide, 5 × saline sodium citrate, 0.1% Tween-20, 50 μg ml −1 heparin, 500 μg ml −1 yeast tRNA) and followed by hybridization with 0.5 ng μl −1 digoxigenin-labelled antisense RNA probe in HM+ buffer. The probes were detected with alkaline phosphatase-conjugated anti-digoxigenin antibodies (1/5,000; Roche Applied Science) using nitro blue tetrazolium chloride/5-bromo-4-chloro-3-indolyl-phosphate, toluidine-salt (Roche Applied Science). After staining embryos were mounted in 90% glycerol prior imaging. Zebrafish Mmp-9 and 13a plasmids were gifts from L. Ramakrishnan laboratory, mmp-2 from A. Noel laboratory. For immunostaining, embryos were incubated with anti-L-plastin antibody (1/10,000, gift from M. Redd), followed by Alexa Fluor 488 Goat Anti-Rabbit IgG antibody (1/1,000, Life Technologies). In vivo zymography In vivo zymography was performed according to Crawford’s protocol [30] . FITC conjugated gelatin (Gelatin-FITC, Anaspec) 1 mg ml −1 in PBS was injected (4–8 ng) into muscle between somite 4 and 5 at 42 h.p.f. Imaging was performed just after injections. Control embryos were either incubated with MMP inhibitors during 4 h prior injections or injected with L-clodronate 17 h prior Gelatin-FITC injections. Statistical analysis Normal distributions were analysed using Shapiro–Wilk test. Non-gaussian data were analysed using Wilcoxon or Kruskal–Wallis test, Gaussian with Student’s t -test or analysis of variance followed by Holm’s multiple comparison. P <0.05 was considered as statistically significant (symbols: *** P <0.001; ** P <0.01; * P <0.05). Statistical analyses were performed using R software. How to cite this article : Travnickova, J. et al . Primitive macrophages control HSPC mobilization and definitive haematopoiesis. Nat. Commun. 6:6227 doi: 10.1038/ncomms7227 (2015).